The miRNA-212/132 family regulates both cardiac hypertrophy and cardiomyocyte autophagy Pathological growth of cardiomyocytes (hypertrophy) is a major determinant for the development of heart failure, one of the leading medical causes of mortality worldwide. Here we show that the microRNA (miRNA)-212/132 family regulates cardiac hypertrophy and autophagy in cardiomyocytes. Hypertrophic stimuli upregulate cardiomyocyte expression of miR-212 and miR-132, which are both necessary and sufficient to drive the hypertrophic growth of cardiomyocytes. MiR-212/132 null mice are protected from pressure-overload-induced heart failure, whereas cardiomyocyte-specific overexpression of the miR-212/132 family leads to pathological cardiac hypertrophy, heart failure and death in mice. Both miR-212 and miR-132 directly target the anti-hypertrophic and pro-autophagic FoxO3 transcription factor and overexpression of these miRNAs leads to hyperactivation of pro-hypertrophic calcineurin/NFAT signalling and an impaired autophagic response upon starvation. Pharmacological inhibition of miR-132 by antagomir injection rescues cardiac hypertrophy and heart failure in mice, offering a possible therapeutic approach for cardiac failure. Heart failure is one of the leading pathological causes of mortality worldwide. Myocardial stress due to injury, valvular heart disease or prolonged hypertension induces pathological hypertrophy, which contributes to the development of heart failure and sudden cardiac death. Initially, cardiac hypertrophy is a compensatory mechanism aiming to decrease wall stress and to increase cardiac output. However, prolonged cardiac hypertrophy progresses to contractile dysfunction, cardiac decompensation and finally to heart failure [1] , [2] . One of the major pathways regulating cardiac hypertrophy involves the anti-hypertrophic FoxO transcription factors, which suppress pro-hypertrophic calcineurin/NFAT signalling [3] , [4] , [5] . In addition, FoxO transcription factors induce apoptosis and autophagy in cardiomyocytes [3] . Autophagy is a catabolic process initiated upon starvation, cellular stress, reactive oxygen species, or accumulation of damaged organelles or protein aggregates. Recent findings suggest a role for autophagy in the maintenance of cardiac homeostasis [6] . Autophagic elimination of damaged organelles, especially mitochondria, is crucial for proper heart function, whereas exaggerated autophagic activity may foster heart failure development [7] . Cardiac-specific loss of autophagy also causes cardiomyopathy in mice [8] . Therefore, a delicate balance of autophagy maintains cardiac homeostasis, whereas the imbalance leads to the progression of heart failure [9] . MicroRNAs (miRNAs) are endogenous small RNA molecules, which regulate their target gene expression post-transcriptionally [10] , [11] . In mice, heart-specific loss-of-function of Dgcr8 or Dicer, key enzymes of the miRNA biogenesis pathway, leads to premature death because of cardiomyopathy associated with myofibrial disarray, fibrosis and ventricular dysfunction [12] , [13] , [14] . However, to date, the functional roles of only few individual miRNAs were shown during heart development or for cardiac homeostasis [15] , [16] , [17] , [18] , [19] , [20] , [21] . Therefore, the generation of loss-of- and gain-of-function mutants for other individual miRNAs is necessary to gain further mechanistic insight into miRNA-dependent regulation of cardiac function and homeostasis. Here we show that hypertrophic conditions induce the expression of miR-212/132 family in cardiomyocytes, and both miR-212 and miR-132 regulate cardiac hypertrophy and cardiomyocyte autophagy. Moreover, pharmacological inhibition of miR-132 by antagomir injection effectively rescues cardiac hypertrophy and heart failure in mice, offering a possible therapeutic approach for cardiac failure. MiR-212/132 family regulates cardiomyocyte hypertrophy We have previously shown upregulation of individual miRNAs in failing mouse and human hearts [22] , [23] , [24] , [25] . However, the functional significance of many miRNAs in heart disease is still not well understood. To determine pro-hypertrophic miRNAs in cardiomyocytes, we transfected neonatal rat cardiomyocytes with a precursor-miRNA library and studied in parallel changes in cardiomyocyte size and secretion of brain natriuretic peptide (BNP). By using a threshold of more than 20% cardiomyocyte size induction, we identified 26 cardiomyocyte-expressed pro-hypertrophic miRNAs, of which ten miRNAs also induced a strong secretion of the cardiac stress marker BNP. The strongest effect on cardiomyocyte hypertrophy was seen after overexpression of miR-212, which together with miR-132 comprises the evolutionary conserved miR-212/132 family ( Fig. 1a ). 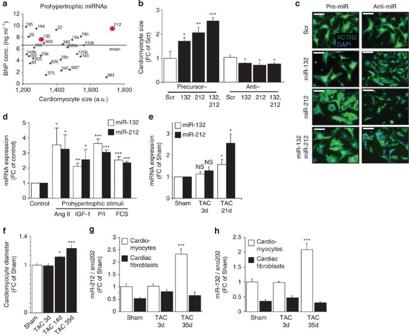Figure 1: MiR-212 and miR-132 are pro-hypertrophic miRNAs induced by hypertrophic stimuli. (a) Overexpression of miRNA precursors from a library identified miRNAs enhancing cardiomyocyte growth and brain natriuretic peptide (BNP) secretion. The miRNA family, miR-212/132, is highlighted by red circles. (b,c) Effects of miR-212 and miR-132 precursors and inhibitors (anti) on cardiomyocyte cell size as compared with the effects of scrambled (Scr) controls (n=5–13). Representative images used for quantification of cardiomyocyte cell size are shown inc. (d) Effects of various pro-hypertrophic stimuli on miR-212 and miR-132 expression in neonatal cardiomyocytes (n=6–10). (e) miR-212 and miR-132 expression levels during pressure-induced left ventricular hypertrophy 3 and 21 days after transaortic constriction (TAC) surgery of mice (n=4). (f) Cardiomyocyte diameters after Sham operation or 3, 14 and 35 days after TAC (n=4 per group). (g,h) miR-212 and miR-132 expression (normalized to sno-202 levels) in fractionated cardiomyocytes and cardiac fibroblasts derived from adult mice after 3 and 35 days of TAC. All values represent mean±s.e.m. *P<0.05; **P<0.01; ***P<0.005. Scale bar increpresents 50 μm. ACTN2, α-cardiac actinin; Ang II, angiotensin-2; a.u., arbitrary unit; d, day; DAPI, 4′,6-diamidino-2-phenylindole; FC, fold change; NS, no significant difference; P/I, phenylephrine/isoprenaline. Figure 1: MiR-212 and miR-132 are pro-hypertrophic miRNAs induced by hypertrophic stimuli. ( a ) Overexpression of miRNA precursors from a library identified miRNAs enhancing cardiomyocyte growth and brain natriuretic peptide (BNP) secretion. The miRNA family, miR-212/132, is highlighted by red circles. ( b , c ) Effects of miR-212 and miR-132 precursors and inhibitors (anti) on cardiomyocyte cell size as compared with the effects of scrambled (Scr) controls ( n =5–13). Representative images used for quantification of cardiomyocyte cell size are shown in c . ( d ) Effects of various pro-hypertrophic stimuli on miR-212 and miR-132 expression in neonatal cardiomyocytes ( n =6–10). ( e ) miR-212 and miR-132 expression levels during pressure-induced left ventricular hypertrophy 3 and 21 days after transaortic constriction (TAC) surgery of mice ( n =4). ( f ) Cardiomyocyte diameters after Sham operation or 3, 14 and 35 days after TAC ( n =4 per group). ( g , h ) miR-212 and miR-132 expression (normalized to sno-202 levels) in fractionated cardiomyocytes and cardiac fibroblasts derived from adult mice after 3 and 35 days of TAC. All values represent mean±s.e.m. * P <0.05; ** P <0.01; *** P <0.005. Scale bar in c represents 50 μm. ACTN2, α-cardiac actinin; Ang II, angiotensin-2; a.u., arbitrary unit; d, day; DAPI, 4′,6-diamidino-2-phenylindole; FC, fold change; NS, no significant difference; P/I, phenylephrine/isoprenaline. Full size image Based on these results, we then focused on the cardiac function of the miR-212/132 family. Validation experiments confirmed that overexpression of either pre-miR-212 or pre-miR-132 leads to cell size enlargement in both primary neonatal cardiomyocytes ( Fig. 1b,c ) and cardiomyocyte cell lines (H9c2, HL-1) ( Supplementary Fig. S1a,d ), indicating that both miR-212 and miR-132 are independently sufficient to induce hypertrophy. Knockdown of these miRNAs with specific miRNA inhibitors in both primary cardiomyocytes and cardiomyocyte cell lines decreased the cell size ( Fig. 1b,c ; Supplementary Fig. S1b,e ), indicating that they are not only sufficient but also required for the physiological enlargement of cardiomyocytes. Expression levels of both miR-212 and miR-132 were upregulated in primary cardiomyocytes upon treatment with different hypertrophic stimuli, such as angiotensin-2, insulin-like growth factor-1 (IGF-1), phenylephrine (PE)/isoprenaline and fetal calf serum (FCS), suggesting that miR-212/132 family is functionally involved in hypertrophic processes induced by different pro-hypertrophic pathways in vitro ( Fig. 1d ). To determine whether miR-212/132 expression would be upregulated in hypertrophic conditions in vivo , we induced cardiac stress in wild-type mice via transaortic constriction (TAC) and showed that cardiac levels of both miR-212 and miR-132 are increased during cardiac hypertrophy ( Fig. 1e ). Of note, this upregulation paralleled the development of cardiac hypertrophy, which is evident by the increase of cardiomyocyte diameter in these hearts ( Fig. 1f ). Importantly, cell fractionation experiments using hearts of Sham- and TAC-operated mice (5 weeks post-TAC) showed that this hypertrophy-induced upregulation of miR-212/132 is observed in cardiomyocytes, but not in cardiac fibroblasts ( Fig. 1g,h ). Taken together, these results demonstrate that miR-212/132 expression is upregulated in cardiomyocytes during hypertrophy both in vitro and in vivo , and both miRNAs are necessary and sufficient for cardiomyocyte hypertrophy in vitro . To further study miR-212/132 functions in cardiomyocytes, we generated H9c2 transgenic cell lines overexpressing miR-212/132 (about tenfold increase; Supplementary Fig. S2a ). In these transgenic cell lines, overexpression of miR-212/132 increased average cell size ( Supplementary Fig. S1c ) and the growth rate in culture ( Supplementary Fig. S2b ). To investigate the cause of higher growth rates, we analysed the levels of proliferation and apoptosis in these cells. Compared with controls, the overexpression of miR-212/132 led to a decrease in apoptosis under both low- and high-FCS conditions ( Supplementary Fig. S2c ), but did not affect cell proliferation ( Supplementary Fig. S2d ). These results demonstrate that miR-212/132 family regulates both apoptosis and hypertrophic growth of cardiomyocytes in vitro . MiR-212/132 overexpression induces cardiac hypertrophy To elucidate whether miR-212/132 overexpression is sufficient to induce cardiac hypertrophy in vivo , we generated transgenic mouse lines with cardiomyocyte-specific overexpression of miR-212/132 under the control of α-myosin heavy chain (MHC) promoter ( Fig. 2a ). We obtained and analysed two independent transgenic lines (Fam23 and Fam43). The overexpression of miR-212 and miR-132 in heart tissues was verified by reverse transcription PCR (RT–PCR) analyses of the mature forms of these miRNAs ( Fig. 2b ). The transgenic mice exhibited no obvious defects at birth. However, the life expectancy was reduced to an average of 84 and 119 days for Fam23 and Fam43, respectively ( Fig. 2c ), and all transgenic mice died with clinical signs of severe heart failure. Explanted hearts from transgenic mice were significantly enlarged ( Fig. 2d ). The heart-to-body-weight ratios of transgenic mice at different ages showed progressive increase of heart mass during adolescence ( Fig. 2e ; Supplementary Fig. S3a ). The expression levels of cardiac stress markers atrial natriuretic peptide (ANP) and BNP were dramatically increased in transgenic hearts ( Supplementary Fig. S3b,c ), indicating development of heart failure. Although the α-MHC levels were not altered, the β-MHC levels were strongly increased in transgenic hearts ( Supplementary Fig. S3d,e ), indicating the 'fetal' gene program reactivation and pathological cardiac remodelling. We also observed increased phospho-Akt levels in miR-212/132-overexpressing transgenic hearts ( Supplementary Fig. S3f ). However, this is probably due to the developing cardiac hypertrophy rather than being the direct consequence of miR-212/132 overexpression, as phospho-Akt levels were unchanged in miR-212/132-overexpressing H9c2 cells in vitro ( Supplementary Fig. S3g ). Morphologically, cardiomyocyte diameter as determined in histological sections of transgenic hearts versus controls, was significantly increased ( Fig. 2f ). Cardiac function in transgenic and wild-type mice was evaluated by small-animal echocardiography. We observed significant end-systolic and end-diastolic left ventricular dilatation in transgenic animals ( Fig. 2g,h ). Fractional shortening, a parameter of cardiac function, was strongly reduced in transgenic mice ( Fig. 2i ). Basic hemodynamic evaluations also confirmed impaired heart function of transgenic animals ( Supplementary Table S1 ). Taken together, these results demonstrate that the cardiomyocyte-specific overexpression of miR-212/132 family in mice is sufficient to induce pathological cardiac hypertrophy resulting in heart failure development. 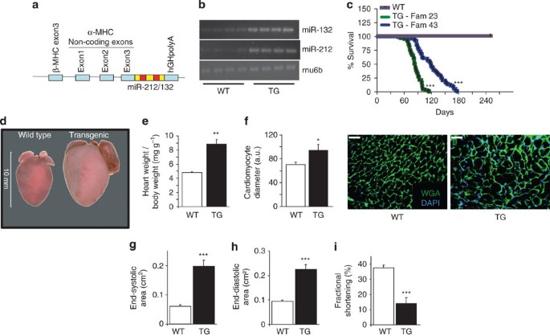Figure 2: Overexpression of miR-212 and miR-132 in cardiomyocytes causes hypertrophy and heart failure. (a) Overexpression construct of miR-212/132 under the control of the α-MHC promoter. (b) Expression levels of miR-212 and miR-132 in heart samples of individual wild-type (WT) and miR-212/132 transgenic (TG) mice as assayed by RT–PCR analysis against the mature forms of corresponding microRNAs. Rnu6b was used as housekeeping control. (c) Survival rate of two different miR-212/132 TG mouse families (TG-Fam23, TG-Fam43) versus WT controls was analysed by Kaplan–Meier survival assay (n=87, 65 and 53 for WT, TG-Fam23 and TG-Fam43, respectively). (d) Morphology of explanted hearts from TG and WT mice at 10 weeks after birth. Scale bar, 1 cm. (e,f) Heart-to-body-weight ratios (e) and cardiomyocyte diameter (f) in 8-week-old α-MHC-miR-212/132 transgenic mice compared with their wild-type littermates (n=5–7). Scale bar, 50 μm. (g–i) Echocardiographic analysis of cardiac dimensions and function for α-MHC-miR-212/132 TG mice and WT controls (n=16–18) (g) end-systolic area, (h) end-diastolic area, (i) fractional shortening. All values ine–irepresent mean±s.e.m. *P<0.05; **P<0.01; ***P<0.005. DAPI, 4′,6-diamidino-2-phenylindole; WGA, wheat germ agglutinin (membrane stain). Figure 2: Overexpression of miR-212 and miR-132 in cardiomyocytes causes hypertrophy and heart failure. ( a ) Overexpression construct of miR-212/132 under the control of the α-MHC promoter. ( b ) Expression levels of miR-212 and miR-132 in heart samples of individual wild-type (WT) and miR-212/132 transgenic (TG) mice as assayed by RT–PCR analysis against the mature forms of corresponding microRNAs. Rnu6b was used as housekeeping control. ( c ) Survival rate of two different miR-212/132 TG mouse families (TG-Fam23, TG-Fam43) versus WT controls was analysed by Kaplan–Meier survival assay ( n =87, 65 and 53 for WT, TG-Fam23 and TG-Fam43, respectively). ( d ) Morphology of explanted hearts from TG and WT mice at 10 weeks after birth. Scale bar, 1 cm. ( e , f ) Heart-to-body-weight ratios ( e ) and cardiomyocyte diameter ( f ) in 8-week-old α-MHC-miR-212/132 transgenic mice compared with their wild-type littermates ( n =5–7). Scale bar, 50 μm. ( g – i ) Echocardiographic analysis of cardiac dimensions and function for α-MHC-miR-212/132 TG mice and WT controls ( n =16–18) ( g ) end-systolic area, ( h ) end-diastolic area, ( i ) fractional shortening. All values in e – i represent mean±s.e.m. * P <0.05; ** P <0.01; *** P <0.005. DAPI, 4′,6-diamidino-2-phenylindole; WGA, wheat germ agglutinin (membrane stain). Full size image To investigate the potentially conserved in vivo roles of miR-212/132 family, we injected miR-212 and miR-132 precursors into zebrafish embryos. Forty-eight hours post-fertilization these embryos showed massive cardiac oedema indicating cardiac dysfunction ( Supplementary Fig. S3h ). These results point to an evolutionary conserved role of miR-212/132 family in the regulation of cardiac function. MiR-212/132 is required for cardiac hypertrophy in mice We previously generated a loss-of-function mutant mouse line for miR-212/132 and demonstrated that female miR-212/132 −/− mice showed an impaired mammary gland development [26] , [27] . We now further analysed the miR-212/132 −/− mouse line to determine whether miR-212/132 is also 'necessary' for either the physiological heart growth or the pathological cardiac hypertrophy. The heart-to-body-weight ratio of adult miR-212/132 −/− mice was 12.3% smaller than their wild-type littermates ( Fig. 3a ), indicating the requirement for miR-212/132 function for proper physiological heart growth. Indeed, isolated primary cardiomyocytes from neonatal miR-212/132 −/− mice had smaller cell sizes compared with that from wild-type littermate controls ( Fig. 3b ). However, cardiac parameters of miR-212/132 −/− mice were absolutely normal ( Supplementary Table S2 ). 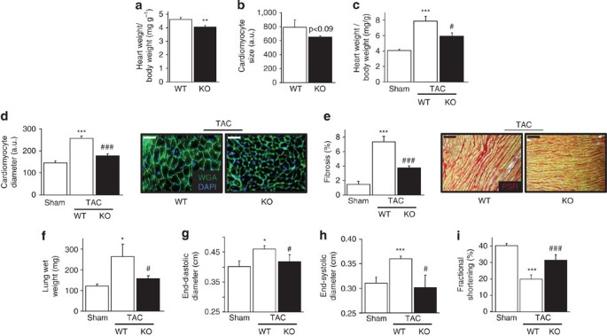Figure 3: MiR-212/132 null mice are protected from transaortic constriction (TAC)-induced hypertrophy and heart failure. (a) Heart-to-body-weight ratios for 12-week-old miR-212/132 null (KO) and wild-type (WT) mice (n=5–6). (b) Cardiomyocyte cell size of neonatal miR-212/132 null and WT mice (n=5–6 isolations). (c–f) Heart-to-body-weight ratios (c), cardiomyocyte diameter (d), cardiac fibrosis (e) and lung wet weight (f) in Sham-operated WT mice and miR-212/132 null and WT mice 3 weeks after TAC surgery (n=4–7). Scale bar, 50 μm. (g–i) Echocardiographic analysis of cardiac dimensions and function in Sham-operated WT mice and miR-212/132 null and WT mice 3 weeks after TAC (n=4–11). (g) End-diastolic area, (h) end-systolic area and (i) fractional shortening. All values represent mean±s.e.m. *P<0.05; **P<0.01; ***P<0.005;#P<0.05 compared with WT TAC;###P<0.005 compared with WT TAC; PSR, picrosirius red (collagen stain). DAPI, 4′,6-diamidino-2-phenylindole; WGA, wheat germ agglutinin. Figure 3: MiR-212/132 null mice are protected from transaortic constriction (TAC)-induced hypertrophy and heart failure. ( a ) Heart-to-body-weight ratios for 12-week-old miR-212/132 null (KO) and wild-type (WT) mice ( n =5–6). ( b ) Cardiomyocyte cell size of neonatal miR-212/132 null and WT mice ( n =5–6 isolations). ( c – f ) Heart-to-body-weight ratios ( c ), cardiomyocyte diameter ( d ), cardiac fibrosis ( e ) and lung wet weight ( f ) in Sham-operated WT mice and miR-212/132 null and WT mice 3 weeks after TAC surgery ( n =4–7). Scale bar, 50 μm. ( g – i ) Echocardiographic analysis of cardiac dimensions and function in Sham-operated WT mice and miR-212/132 null and WT mice 3 weeks after TAC ( n =4–11). ( g ) End-diastolic area, ( h ) end-systolic area and ( i ) fractional shortening. All values represent mean±s.e.m. * P <0.05; ** P <0.01; *** P <0.005; # P <0.05 compared with WT TAC; ### P <0.005 compared with WT TAC; PSR, picrosirius red (collagen stain). DAPI, 4′,6-diamidino-2-phenylindole; WGA, wheat germ agglutinin. Full size image To determine whether miR-212/132 family is required for pathological cardiac hypertrophy, we applied left ventricular pressure overload by TAC operation to miR-212/132 −/− mice and their wild-type littermates. TAC led to a significant increase in cardiac weight and cross-sectional cardiomyocyte diameters in wild-type animals ( Fig. 3c,d ). In contrast, miR-212/132 −/− mice were protected from TAC-induced hypertrophy ( Fig. 3c,d ). TAC-induced cardiac fibrosis was less in mutant hearts ( Fig. 3e ). Increase in lung weight was blunted in miR-212/132 −/− mice compared with wild-type littermates, indicating prevention of heart failure ( Fig. 3f ). Three weeks after TAC, wild-type mice developed left ventricular dilatation and impaired cardiac function as shown by increased end-diastolic and end-systolic diameters and decreased fractional shortening ( Fig. 3g–i ). By contrast, miR-212/132 −/− mice were partially protected from development of cardiac dilatation and impaired left ventricular function ( Fig. 3g–i ). These results demonstrate that miR-212/132 family is not only 'sufficient' to induce cardiac hypertrophy, but also 'necessary' for both physiological and pathological hypertrophy in vivo . As miR-212/132 −/− mice bear constitutive deletion of miR-212/132 , we also investigated the potential impacts of miR-212/132 loss-of-function in non-cardiomyocyte cells of the heart. We knocked-down miR-132 and/or miR-212 in cardiac fibroblasts, the major cell fraction of cardiac non-myocytes, but did not observe any phenotypic effect on their proliferation, apoptosis or migratory behaviour ( Supplementary Fig. S4 ). Next, to identify potential miR-212/132 loss-of-function phenotypes in general angiogenesis in vivo , we used a retinal angiogenesis assay using wild-type and miR-212/132 −/− mice but observed no differences in retinal area, number of retinal arteries, central retinal artery diameter or number of branches per area ( Supplementary Fig. S5a–c ). Furthermore, we analysed capillary densities in wild-type and miR-212/132 −/− hearts but found no significant differences ( Supplementary Fig. S5d ). Taken together, we concluded that the observed cardio-protective phenotype in miR-212/132 −/− mice is likely due to the miR-212/132 loss-of-function in cardiomyocytes rather than in non-cardiomyocyte cells of the heart. MiR-212 and miR-132 directly regulate FoxO3 expression To elucidate the molecular functions of miR-212/132 family in the regulation of cardiac hypertrophy, we screened predicted target genes for both miRNAs in silico to identify hypertrophy-associated putative target genes. Interestingly, the anti-hypertrophic transcription factor FoxO3 was a predicted target of both miR-212 and miR-132. To validate this bioinformatic prediction, we cloned the 3′ untranslated region (3′UTR) of FoxO3 downstream of the firefly luciferase gene and found that the normalized luciferase activity was substantially reduced upon cotransfection of this construct with either miR-212 or miR-132 but not with unrelated control (scrambled) miRNA ( Fig. 4a ). Mutation of the miR-212- and miR-132-binding sites within the FoxO3 3′UTR abolished the repressing effects of miR-212 and miR-132 ( Fig. 4a ). These results validate FoxO3 as a direct target of both miR-212 and miR-132. 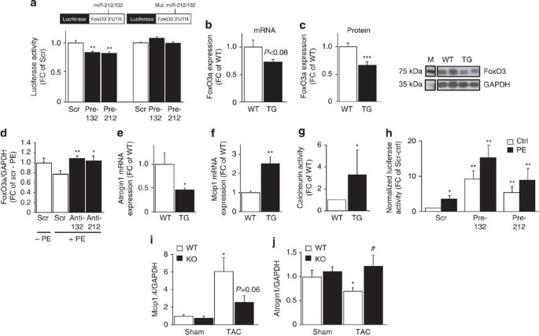Figure 4: MiR-212 and miR-132 regulate calcineurin signalling via targeting FoxO3 expression. (a) Luciferase activity levels upon cotransfection of a luciferase construct containing wild-type (WT) or mutated (Mut.) 3′UTR ofFoxO3with scrambled (Scr) control (Ctrl), pre-miR-132 or pre-miR-212 (n=9). (b,c) Expression levels of FoxO3 on mRNA (b) and protein levels (c) in hearts of WT and α-MHC-miR-212/-132 transgenic (TG) mice. M: Size marker (n=9–13). (d) FoxO3 mRNA levels in neonatal rat cardiomyocytes transfected with Scr Ctrl, anti-miR-212 and anti-miR-132 after phenylephrine (PE, 10 μM) treatment (n=6–9;P-values against Scr+PE). (e–g) Expression levels of atrogin-1 (e) and Mcip1 (f) and calcineurin phosphatase activity levels (g) in hearts of WT and α-MHC-miR-212/132 TG mice (n=5–9). (h) Luciferase activity levels showing the NFAT transcriptional activity in cardiomyocytes transfected with Scr Ctrl, pre-miR-132 or pre-miR-212 (n=5). (i,j) Mcip1.4 (i) and atrogin-1 (j) mRNA levels in WT and miR-212/132 null (KO) mice 3 weeks after transaortic constriction (TAC) or Sham operation (n=5–7 per group). All values represent mean±s.e.m. *P<0.05; **P<0.01; ***P<0.005.#P<0.05 compared with WT TAC. FC, fold change. Figure 4: MiR-212 and miR-132 regulate calcineurin signalling via targeting FoxO3 expression. ( a ) Luciferase activity levels upon cotransfection of a luciferase construct containing wild-type (WT) or mutated (Mut.) 3′UTR of FoxO3 with scrambled (Scr) control (Ctrl), pre-miR-132 or pre-miR-212 ( n =9). ( b , c ) Expression levels of FoxO3 on mRNA ( b ) and protein levels ( c ) in hearts of WT and α-MHC-miR-212/-132 transgenic (TG) mice. M: Size marker ( n =9–13). ( d ) FoxO3 mRNA levels in neonatal rat cardiomyocytes transfected with Scr Ctrl, anti-miR-212 and anti-miR-132 after phenylephrine (PE, 10 μM) treatment ( n =6–9; P -values against Scr+PE). ( e – g ) Expression levels of atrogin-1 ( e ) and Mcip1 ( f ) and calcineurin phosphatase activity levels ( g ) in hearts of WT and α-MHC-miR-212/132 TG mice ( n =5–9). ( h ) Luciferase activity levels showing the NFAT transcriptional activity in cardiomyocytes transfected with Scr Ctrl, pre-miR-132 or pre-miR-212 ( n =5). ( i , j ) Mcip1.4 ( i ) and atrogin-1 ( j ) mRNA levels in WT and miR-212/132 null (KO) mice 3 weeks after transaortic constriction (TAC) or Sham operation ( n =5–7 per group). All values represent mean±s.e.m. * P <0.05; ** P <0.01; *** P <0.005. # P <0.05 compared with WT TAC. FC, fold change. Full size image We then analysed FoxO3 levels in transgenic hearts and found a reduced expression both at mRNA and protein levels compared with wild-type hearts ( Fig. 4b,c ). MiR-212/132 overexpression also resulted in lower FoxO3 levels in H9c2 and primary cardiomyocytes ( Supplementary Fig. S6a,b ). PE treatment-induced FoxO3 downregulation in cardiomyocytes was rescued upon inhibition of miR-212 or miR-132 ( Fig. 4d ), indicating that hypertrophy-induced FoxO3 downregulation is indeed mediated by the miR-212/132 family. As FoxO3 downregulation is also associated with human heart failure [22] , this finding represents a remarkable similarity of the observed phenotype in our transgenic mouse line to human heart failure also at a molecular level. FoxO transcription factors exert their anti-hypertrophic functions largely via the suppression of the calcineurin signalling [3] , [4] . FoxO3 can activate the expression of atrogin-1, which induces the ubiquitination and thus degradation of calcineurin-A in cardiomyocytes [28] , [29] . Therefore, we analysed atrogin-1 expression levels in transgenic hearts and found a significant reduction compared with wild-type hearts ( Fig. 4e ). Because of the miR-212/132-dependent downregulation of FoxO3 and subsequently that of atrogin-1 expression, we hypothesized that the calcineurin activity would be increased in transgenic hearts. We thus analysed mRNA levels of Mcip1, a direct transcriptional target of the calcineurin signalling [30] , and found a significant increase in transgenic hearts ( Fig. 4f ), as well as in the miR-212/132-overexpressing transgenic H9c2 cells ( Supplementary Fig. S6c ). Moreover, increased calcineurin phosphatase activity was detected in transgenic hearts, thus confirming the hyperactivity of this pro-hypertrophic signalling pathway ( Fig. 4g ). The pro-hypertrophic effect of the calcineurin signalling is mainly mediated by activation of the nuclear factor of activated T-cells (NFAT) transcription factors [2] , [31] . Therefore, we also analysed NFAT transcriptional activity levels in cardiomyocytes after transfection with pre-miR-212 or pre-miR-132. Overexpression of either miR-212 or miR-132, but not the control miRNA, led to a dramatic increase in NFAT activity both in basal and PE-induced pro-hypertrophic conditions ( Fig. 4h ). In miR-212/132 −/− hearts, Mcip1.4 upregulation after pressure overload was attenuated ( Fig. 4i ), indicating that miR-212/132 is required for the activation of the calcineurin/NFAT signalling during pressure-overload-induced cardiac hypertrophy. In addition, atrogin-1 downregulation observed in wild-type hearts during cardiac hypertrophy was blunted in miR-212/132 −/− hearts ( Fig. 4j ), indicating the unsuppressed FoxO3 function and thereby explaining the attenuated calcineurin signalling in miR-212/132 −/− hearts after pressure overload. Taken together, these results indicate that miR-212/132 family regulates hypertrophic pathways in cardiomyocytes via direct downregulation of FoxO3 expression. In the absence of FoxO3-mediated inhibition, the hyperactivation of the calcineurin/NFAT signalling pathway probably leads to the observed pathological hypertrophy and the associated heart failure in the miR-212/132-overexpressing transgenic mice. Conversely, in miR-212/132 −/− hearts after pressure overload, the unsuppressed FoxO3 activity leads to the upregulation of atrogin-1 and thereby prevents the activation of the calcineurin signalling and thus development of cardiac hypertrophy. MiR-212/132 regulates autophagy in cardiomyocytes FoxO3 is also an important pro-autophagic factor in cardiomyocytes [32] , [33] . To determine whether miR-212/132 overexpression in cardiomyocytes might interfere with autophagic processes in vivo , we investigated the expression of several autophagic marker genes and found a dramatic decrease in their expression in transgenic hearts ( Fig. 5a ). Likewise, the LC3 lipidation levels (LC3II/LC3I ratios) were lower ( Fig. 5b ), whereas autophagy substrate p62 levels were increased in miR-212/132-overexpressing transgenic hearts ( Fig. 5c ). These results suggest that cardiomyocyte-specific miR-212/132-overexpression attenuates cardiac autophagic processes. Conversely, miR-212/132 −/− hearts had higher cardiac LC3 lipidation and lower p62 levels compared with wild-type hearts ( Fig. 5b,c ), indicating higher rates of autophagy. 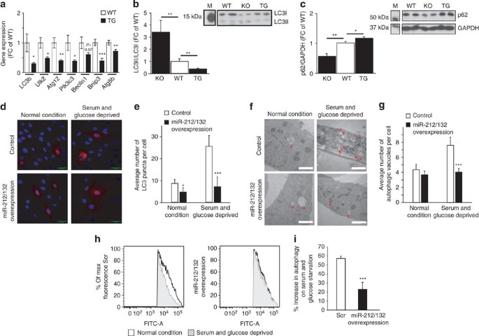Figure 5: MiR-212 and miR-132 are anti-autophagic factors in cardiomyocytes. (a) mRNA expression levels of autophagic marker genes in hearts of wild-type (WT) and α-MHC-miR-212/132 transgenic (TG) mice (n=9–10). (b,c) Ratio of LC3II to LC3I (b) and p62 protein levels (c) in WT, miR-212/132 null (KO) and α-MHC miR-212/132 TG mice. M: Size marker (n=4–12). (d,e) Representative images (d) and quantification (e) of LC3:mCherry puncta (in red) in control and miR-212/132-overexpressing TG H9c2 cells under normal and serum/glucose-deprivation conditions (n=30). Nuclei are stained in blue with Hoechst33342. (f,g) Representative electron microscopy images (f) and quantification (g) of autophagic vacuoles in control and miR-212/132-overexpressing TG H9c2 cells under normal and serum/glucose-deprivation conditions (n=20). (h,i) Representative FACS plots (h) and quantification (i) of percent increase of autophagic flux in control and miR-212/132-overexpressing TG H9c2 cells under normal and serum/glucose-deprivation conditions (n=3–4 experiments). All values represent mean±s.e.m. *P<0.05; **P<0.01; ***P<0.005. Scale bars, 50 μm indand 2 μm inf. FC, fold change. Figure 5: MiR-212 and miR-132 are anti-autophagic factors in cardiomyocytes. ( a ) mRNA expression levels of autophagic marker genes in hearts of wild-type (WT) and α-MHC-miR-212/132 transgenic (TG) mice ( n =9–10). ( b , c ) Ratio of LC3II to LC3I ( b ) and p62 protein levels ( c ) in WT, miR-212/132 null (KO) and α-MHC miR-212/132 TG mice. M: Size marker ( n =4–12). ( d , e ) Representative images ( d ) and quantification ( e ) of LC3:mCherry puncta (in red) in control and miR-212/132-overexpressing TG H9c2 cells under normal and serum/glucose-deprivation conditions ( n =30). Nuclei are stained in blue with Hoechst33342. ( f , g ) Representative electron microscopy images ( f ) and quantification ( g ) of autophagic vacuoles in control and miR-212/132-overexpressing TG H9c2 cells under normal and serum/glucose-deprivation conditions ( n =20). ( h , i ) Representative FACS plots ( h ) and quantification ( i ) of percent increase of autophagic flux in control and miR-212/132-overexpressing TG H9c2 cells under normal and serum/glucose-deprivation conditions ( n =3–4 experiments). All values represent mean±s.e.m. * P <0.05; ** P <0.01; *** P <0.005. Scale bars, 50 μm in d and 2 μm in f . FC, fold change. Full size image To determine whether attenuated autophagy in transgenic hearts is a direct effect of miR-212/132 overexpression, we further analysed autophagic processes in miR-212/132-overexpressing transgenic H9c2 cells. To visualize autophagic structures in cardiomyocytes, we transfected them with an expression construct for LC3:mCherry fusion protein, which allows the visualization of autophagic structures as fluorescent puncta [34] . Under normal conditions, the average number of LC3-puncta was slightly reduced in miR-212/132-overexpressing H9c2 cells in comparison to controls ( Fig. 5d,e ). After induction of autophagic conditions by starving these cells in serum/glucose-free media [35] , the average number of LC3-puncta increased threefold in control cells, but was almost unchanged in miR-212/132-overexpressing transgenic cells ( Fig. 5d,e ). Similar findings were observed in primary neonatal cardiomyocytes ( Supplementary Fig. S7 ). These results demonstrate that miR-212/132 family negatively regulates the autophagic response of cardiomyocytes to nutrient limitation. We next used transmission electron microscopy for analysing these cells by quantifying the number of autophagic vacuoles. Similar to our findings described above, the autophagic response to nutrient limitation was blunted in miR-212/132-overexpressing H9c2 cells compared with almost twofold increase of the number of autophagic vacuoles in control cells ( Fig. 5f,g ). Finally, for the quantitative detection of autophagic flux, we used a FACS-based method [36] to analyse the transgenic H9c2 cells transfected with GFP:LC3 expression constructs. A significant decrease in GFP intensity was detected for control cells upon starvation, indicating increased autophagic activity. In contrast, for the miR-212/132-overexpressing transgenic H9c2 cells, this decrease in GFP intensity was markedly reduced ( Fig. 5h,i ). Of note, total GFP:LC3 fusion protein levels were similar between control and miR-212/132-overexpressing H9c2 cells under the same experimental conditions ( Supplementary Fig. S8 ). Taken together, our data indicate by three independent methods that miR-212/132 family has an anti-autophagic function in cardiomyocytes, which can blunt the autophagic response to nutrient limitation upon their overexpression. To determine whether our findings demonstrate a biologically relevant mechanism in cardiomyocytes, we analysed miR-212 and miR-132 levels in wild-type H9c2 cells under normal and nutrient-limiting conditions. Our results showed that during nutrient-limiting conditions cardiomyocytes downregulate the expression of the anti-autophagic miR-212/132 family, which might represent a mechanism facilitated by these cells to increase the level of autophagic response to starvation conditions ( Supplementary Fig. S9 ). To study the potential impact of miR-212/132 family on autophagic response to starvation in vivo , we performed starvation experiments using both miR-212/132 loss-of- and gain-of function mutant mouse lines ( Fig. 6a ). As assessed by LC3 lipidation levels, starvation led to a marked increase in cardiac autophagy in wild-type mice, which was significantly attenuated in cardiomyocyte-specific miR-212/132-overexpressing mice ( Fig. 6b ). Interestingly, upon starvation autophagy levels increased to comparable levels in wild-type and miR-212/132 −/− hearts ( Fig. 6b ). To evaluate the autophagic structures on ultrastructural level, we further analysed these heart samples by transmission electron microscopy ( Fig. 6c and Supplementary Fig. S10 ). Under normal 'fed' conditions, we observed more autophagic vacuoles within the cardiomyocytes of miR-212/132 −/− mice than of the wild-type mice, indicating increased basal levels of autophagy. Starvation increased abundance of autophagic vacuoles in wild-type cardiomyocytes, which reached to a similar level of slightly increased autophagic vacuole numbers in starved miR-212/132 −/− cardiomyocytes. On the other hand, in cardiomyocytes of miR-212/132-overexpressing transgenic mice we observed very few autophagic vacuoles and electron-dense autophagosomes under normal conditions, which only slightly increased upon starvation. This result also confirms that levels of both basal and starvation-induced autophagy are blunted in miR-212/132-overexpressing cardiomyocytes. 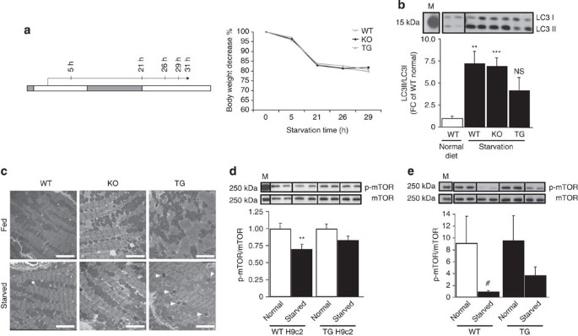Figure 6: MiR-212 and miR-132 inhibit starvation-induced autophagyin vivo. (a) Schematic representation of starvation experiment in mice. The white and grey parts on the time line represent the day and night phases, respectively. The arrow shows the start and duration of the starvation and the indicated time points of starvation are when animals are scored for body conditioning index. (b) LC3II to LC3I ratios in wild-type (WT) mice fed with normal diet and WT, miR-212/132−/−null and α-MHC miR-212/132 transgenic (TG) mice under starvation for 31 h (n=4). (c) Electron micrographs from ultrathin sections of resin-embedded heart biopsies of fed and starved WT, miR-212/132 null (KO) and cardiomyocyte-specific miR-212/132-overexpressing (TG) mice. White spots around the mitochondria (dark grey structures) are autophagic vacuoles. The electron-dense black spots shown with white arrows are autophagosomes. Scale bars, 4 μm. (d) p-mTOR/mTOR ratios in WT and miR-212/132 TG H9c2 cells 24 h after normal and starvation (serum/glucose-deprived) conditions (n=6). (e) p-mTOR/mTOR ratios in hearts of WT and α-MHC miR-212/132 TG mice fed with normal diet or 31 h after starvation (n=4). M, size marker. All values represent mean±s.e.m. **P<0.01; ***P<0.005;#P=0.11. Figure 6: MiR-212 and miR-132 inhibit starvation-induced autophagy in vivo . ( a ) Schematic representation of starvation experiment in mice. The white and grey parts on the time line represent the day and night phases, respectively. The arrow shows the start and duration of the starvation and the indicated time points of starvation are when animals are scored for body conditioning index. ( b ) LC3II to LC3I ratios in wild-type (WT) mice fed with normal diet and WT, miR-212/132 −/− null and α-MHC miR-212/132 transgenic (TG) mice under starvation for 31 h ( n =4). ( c ) Electron micrographs from ultrathin sections of resin-embedded heart biopsies of fed and starved WT, miR-212/132 null (KO) and cardiomyocyte-specific miR-212/132-overexpressing (TG) mice. White spots around the mitochondria (dark grey structures) are autophagic vacuoles. The electron-dense black spots shown with white arrows are autophagosomes. Scale bars, 4 μm. ( d ) p-mTOR/mTOR ratios in WT and miR-212/132 TG H9c2 cells 24 h after normal and starvation (serum/glucose-deprived) conditions ( n =6). ( e ) p-mTOR/mTOR ratios in hearts of WT and α-MHC miR-212/132 TG mice fed with normal diet or 31 h after starvation ( n =4). M, size marker. All values represent mean±s.e.m. ** P <0.01; *** P <0.005; # P =0.11. Full size image Next, we analysed p62 levels under starvation conditions both in vitro and in vivo. Surprisingly, starvation led to p62 upregulation in both wild-type and miR-212/132-overexpressing H9c2 cells, as well as in wild-type and miR-212/132 −/− hearts ( Supplementary Fig. S11 ). By contrast, p62 levels remained unchanged in miR-212/132-overexpressing hearts upon starvation. As p62 regulates the formation of protein aggregates and is removed by autophagy [37] , its levels are in general inversely correlated with the autophagic activity. However, starvation conditions may possibly induce upregulation of p62 expression in cardiomyocytes. Indeed, during myocardial infarction p62 levels were shown to increase in parallel to increased autophagic activity [38] . Autophagic response to nutrient limitation also involves anti-autophagic mTOR activity [39] . We thus analysed phospho-mTOR levels in our samples. In wild-type H9c2 cells, phospho-mTOR/mTOR levels were reduced upon starvation ( Fig. 6d ), thus confirming the increased autophagy in these cells. In contrary, we observed only a slight, but insignificant, decrease in starved miR-212/132-overexpressing H9c2 cells ( Fig. 6d ), supporting our previous finding of blunted autophagic response in these cells. Likewise, although cardiac phospho-mTOR/mTOR levels markedly decreased upon starvation, the level of downregulation was lower in transgenic hearts, thus confirming the attenuated autophagic response phenotype in vivo caused by (or 'due to') miR-212/132 overexpression ( Fig. 6e ). The IGF-1/PI3K pathway and FoxO3 are important regulators of autophagy in cardiomyocytes during starvation [32] , [35] . Here, we demonstrated that miR-212/132 family, which can be upregulated by IGF-1 signalling ( Fig. 1d ) and suppresses FoxO3 expression ( Fig. 4a–c ), negatively regulates the autophagy in cardiomyocytes. In miR-212/132-overexpressing H9c2 cells, less FoxO3 proteins were detected on the LC3 promoter regions ( Supplementary Fig. S12a ), suggesting that the anti-autophagic function of miR-212/132 family is related to miR-212/132-mediated suppression of FoxO3. This was also confirmed by lower LC3b expression in the starving miR-212/132-overexpressing cells ( Supplementary Fig. S12b ). Taken together, our results demonstrate that miR-212/132 acts as an anti-autophagic factor in cardiomyocytes via regulating FoxO3 expression. MiR-212/132 overexpression attenuates the starvation-induced autophagic response in cardiomyocytes both in vitro and in vivo . On the other hand, loss of function of miR-212/132 increases the basal levels of autophagy in the heart. Antagomir-132 injection rescues heart failure in mice Based on the phenotypical observations in gain-of- and loss-of-function studies, we hypothesized that inhibition of either miR-212 or miR-132 using specific antagomirs might prevent the development of pressure-overload-induced heart failure. Towards this aim, we induced cardiac hypertrophy in wild-type mice by TAC and injected specific antagomirs against miR-132 intravenously. Endogenous cardiac miR-132 levels were successfully knocked-down in mice treated with antagomir against miR-132 but not with the control antagomir against a scrambled sequence ( Supplementary Fig. S13 ). Heart-to-body-weight ratios and cardiomyocyte diameters were significantly increased in control-treated animals after pressure overload, but less affected in antagomir-132-treated mice ( Fig. 7a,b ). Antagomir-132-treated mice also showed less increase in cardiac fibrosis ( Fig. 7c ). Moreover, cardiac function and dilatation was better preserved in antagomir-132-treated mice compared with the control-treated group ( Fig. 7d–f ). In hearts of antagomir-132-treated mice, FoxO3 protein levels were higher compared with control treatment ( Fig. 7g ), and the TAC-induced upregulation of calcineurin activity and Mcip1.4 expression were attenuated ( Fig. 7h,i ). Taken together, these results suggest that at least in mice, the antagomir-mediated silencing of miR-132 can be used to prevent the development of cardiac hypertrophy and subsequent heart failure. 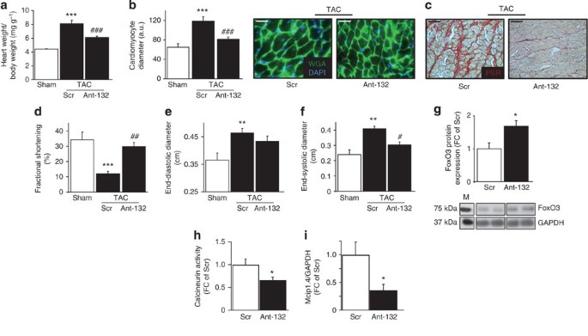Figure 7: Anti-miR-132 therapy prevents pressure-overload-induced heart failure. (a–c) Heart-to-body-weight ratios (a), cardiomyocyte diameters (b) and cardiac fibrosis (c) in Sham-operated mice and mice treated with intravenous injection of either scrambled control (Scr) or miR-132 inhibitors (Ant-132) after TAC. These mice were analysed 3 weeks after TAC (n=4–11). PSR, picrosirius red staining. (d–f) Echocardiographic analysis of cardiac dimensions and function in Sham-operated mice and mice treated with intravenous injection of either control (Scr) or miR-132 inhibitors (Ant-132) after TAC. These mice were analysed 3 weeks after TAC for (d) fractional shortening, (e) end-diastolic area and (f) end-systolic area (n=4–9). (g–i) Cardiac FoxO3 protein levels (g), calcineurin activity (h) and Mcip1.4 mRNA levels (i) in mice treated with intravenous injection of either control (Scr) or miR-132 inhibitors (Ant-132) 3 weeks after TAC and treatment (n=4–8). M: size marker. All values represent mean±s.e.m. *P<0.05; **P<0.01; ***P<0.005;#P<0.05 against TAC-control;##P<0.01 against TAC-control;###P<0.005 against TAC-control. Scale bars, 50 μm. DAPI, 4′,6-diamidino-2-phenylindole; FC, fold change; WGA, wheat germ agglutinin. Figure 7: Anti-miR-132 therapy prevents pressure-overload-induced heart failure. ( a – c ) Heart-to-body-weight ratios ( a ), cardiomyocyte diameters ( b ) and cardiac fibrosis ( c ) in Sham-operated mice and mice treated with intravenous injection of either scrambled control (Scr) or miR-132 inhibitors (Ant-132) after TAC. These mice were analysed 3 weeks after TAC ( n =4–11). PSR, picrosirius red staining. ( d – f ) Echocardiographic analysis of cardiac dimensions and function in Sham-operated mice and mice treated with intravenous injection of either control (Scr) or miR-132 inhibitors (Ant-132) after TAC. These mice were analysed 3 weeks after TAC for ( d ) fractional shortening, ( e ) end-diastolic area and ( f ) end-systolic area ( n =4–9). ( g – i ) Cardiac FoxO3 protein levels ( g ), calcineurin activity ( h ) and Mcip1.4 mRNA levels ( i ) in mice treated with intravenous injection of either control (Scr) or miR-132 inhibitors (Ant-132) 3 weeks after TAC and treatment ( n =4–8). M: size marker. All values represent mean±s.e.m. * P <0.05; ** P <0.01; *** P <0.005; # P <0.05 against TAC-control; ## P <0.01 against TAC-control; ### P <0.005 against TAC-control. Scale bars, 50 μm. DAPI, 4′,6-diamidino-2-phenylindole; FC, fold change; WGA, wheat germ agglutinin. Full size image Here we demonstrate that miR-212/132 family has a key role in cardiac hypertrophy and heart failure development. Both miR-212 and miR-132 are upregulated by cardiac stress in vivo and upon hypertrophic conditions in vitro . Our results show that miR-212 and miR-132 are both necessary and sufficient for pathological hypertrophy of cardiomyocytes in vitro and cardiac hypertrophy in vivo . Transgenic mouse lines with cardiomyocyte-specific miR-212/132 overexpression developed cardiac hypertrophy and subsequent heart failure. Conversely, miR-212/132 −/− mice were protected from pathological cardiac hypertrophy induced by pressure overload. Similarly, pharmacologic inhibition of miR-132 by antagomir injection blocked cardiac hypertrophy and development of heart failure. Our results show that both miR-212 and miR-132 target and negatively regulate the expression of the FoxO3 transcription factor, a powerful anti-hypertrophic and pro-autophagic factor in cardiomyocytes [4] , [32] . The FoxO3 downregulation upon miR-212/132-overexpression results in the hyperactivation of the pro-hypertropic calcineurin/NFAT signalling pathway, which subsequently leads to the hypertrophy of cardiomyocytes. Conversely, the genetic loss-of-function of miR-212/132 or the antagomir-mediated knockdown of miR-132 suppresses the pressure-overload-induced calcineurin/NFAT signalling and thereby attenuates the development of cardiac hypertrophy. Cardiomyocytes are extremely sensitive to nutrient-limitation and facilitate autophagic mechanisms to cope with starvation. We showed that miR-212/132 family has anti-autophagic function in cardiomyocytes and can attenuate this starvation-induced autophagic response upon their overexpression. On the other hand, miR-212/132 −/− mice showed higher levels of basal autophagy under normal conditions. Reduced cardiac autophagy is associated with age-related cardiomyopathy [40] . As miR-212/132 overexpression in cardiomyocytes impairs autophagy and leads to severe heart failure development in mice, the dysfunction of autophagic response mechanisms may possibly also contribute to the observed cardiac death. However, our results do not provide a mechanistic link between autophagy and cardiac hypertrophy, but rather demonstrate two different functions of miR-212/132 family in the heart. MiRNAs can regulate several gene targets simultaneously in a cell. Therefore, we cannot rule out if dysregulation of other, yet unknown miR-212/132 targets also contributed to the observed loss-of- and gain-of-function phenotypes. Although we did not detect any miR-212/132 loss-of-function phenotypes in cardiac fibroblasts in vitro , and in general angiogenesis or cardiac capillary densities in vivo , we cannot completely exclude the possibility that miR-212/132 loss-of-function in non-myocyte cells of the heart also made minor contributions to the observed cardioprotective phenotype in these mice. Nevertheless, as we observed opposite phenotypes in cardiomyocyte-specific miR-212/132-overexpressing transgenic mice and the miR-212/132 −/− mice and experiments using cardiomyocyte cell lines also reproduce the hypertrophy and autophagy phenotypes in vitro , it is highly likely that the cardioprotective phenotype in miR-212/132 −/− mice is due to the miR-212/132 loss-of-function in cardiomyocytes. FoxO3 also regulates miR-1 levels in cardiomyocytes [41] . Indeed, miR-1 levels were downregulated in miR-212/132-overexpressing transgenic hearts and H9c2 cell lines ( Supplementary Fig. S14 ), which may also contribute to the observed heart failure phenotype in the transgenic mice. Despite the development of new therapeutic approaches for heart failure in the last decades, the mortality rates still remain unacceptably high [2] . Thus, there is a great urge to develop more efficient novel therapeutic approaches. Our findings by using intravenous injection of antagomirs against miR-132 offer a promising novel therapeutic approach for pressure-overload-induced heart failure. Furthermore, our findings here represent the first in vivo example of miRNA-regulated autophagy. Cell culture and transfections Primary cardiomyocytes were prepared from neonatal mice or rats using standard protocols. H9c2 cells and primary cardiomyocytes were maintained in DMEM+10% FCS (with exception of the starvation and FCS-mediated hypertrophy experiments). HL1 cells were maintained in Claycomb medium+10% FCS. For both stable and transient transfection of primary cardiomyocytes or cell lines, Lipofectamine 2000 reagent (Invitrogen, Karlsruhe, Germany) was used according to the manufacturer's protocol. For the screen of pro-hypertrophic miRNAs, miRNA precursor library (Pre-miR miRNA Precursor Library–Mouse V3, Ambion; each 50 nM) was used. For measurement of cell size, cells were fixed with 4% paraformaldehyde and surface area of cardiomyocytes was calculated after α-actinin staining (ACTN2; 1:1,000; Sigma, A7811) using the AxioVison Rel 4.4 package (Carl Zeiss). The percentage of cells undergoing apoptosis in cell line cultures was determined by staining with annexin-V and propidium iodide followed by FACS analysis (annexin-V-FLUOS kit, Roche). To measure proliferative capacity in miRNA-modulated cells, a WST-1 proliferation assay (Roche, Germany) was performed according to the manufacturer's protocols. For measuring migratory capacity a defined scratch was created 72 h post transfection and blank distance was measured at 0 h and after 5 h. Migratory index was calculated by using the formula: migratory index=distance (0 h)−distance ( t h)/distance (0 h). To generate stably transfected miR-212/132 overexpressing transgenic H9c2 cell lines, an expression construct was prepared by cloning the whole miR-212/132 genomic locus (3.4 kb) downstream of a cytomegalovirus promoter within the pTARGET vector (Promega). The expression construct used contained a neomycin gene under the control of a PGK promoter. The prepared construct or the original pTARGET vector (as control) was used to transfect cells of the H9c2 cell line. After transfections, cells were cultured in DMEM with 10% FCS and 1 mg ml −1 G418 (Roche) for 8 days. Two independent transfections for both miR-212/132 overexpression construct and the control construct were prepared. After the initial G418-mediated selection, the stably transfected cells were cultured during maintenance and the experiments with 0.5 mg ml −1 of G418. Mouse lines and animal studies All animal studies were performed in accordance with the relevant guidelines and regulations and with the approval of the responsible local and national authorities. MiR-212/132 loss-of-function mutant mouse line was generated previously [26] . This mouse line was backcrossed into C57Bl/6N background for at least seven generations. For the generation of the transgenic mouse lines with the cardiomyocyte-specific overexpression of miR-212/132, a 486-bp genomic region of the miR-212/132 genomic locus, containing the sequences encoding the hairpin-stem loop sequences of both miR-212 and miR-132, was cloned downstream of the third exonic sequence of α-MHC gene and upstream of the hGH polyA signal sequence as shown in Fig. 2a . Linearized construct was microinjected into the pronuclei of fertilized eggs. Two independent founder lines were obtained with the heart-specific overexpression of miR-212/132. Afterwards, both lines were backcrossed into C57BL/6N background for at least six generations. Cardiac dimensions and function were analysed by pulse–wave Doppler echocardiography essentially as described [42] . TAC model and antagomir application TAC was performed on male C57BL/6 mice (10- to 12-week old) from Charles River Laboratories or α-MHC-miR-212/132 transgenic mice or their littermate controls essentially as described [43] . Antagomirs were synthesized as described [44] , and were directed against miR-132 or a scrambled sequence (control). Treatment started during the TAC operation, and animals received control or antagomir-132 injections by retro-orbital injection (day 0 and day 1, 0.1 ml volume containing antagomir-132 or control (each 80 mg kg −1 body weight)). Cardiac cell fractionation Intact hearts were perfused with collagenase-based enzymatic solution (collagenase type II) through the aorta. Thereafter, heart tissue was minced and gently passed through 1 ml syringe for 3 min to produce cell suspensions. Cell fractionation of cardiomyocytes and cardiac fibroblasts were done as described before [24] . Histological analyses of heart samples For analysis of collagen deposition, paraffin sections of the left ventricular myocardium were stained with Sirius red and picric acid. Collagen content was calculated as the percentage of the area in each section that was stained with Sirius red. For capillary counting, sections were stained for Pecam1 (CD31; 1:50; AbD Serotec, MCA2388), 4',6-Diamidino-2-phenylindole and wheat germ agglutinin (1:100; Invitrogen, W11261) and counting was done by NIKON-NIS Element Software. For each animal four to seven regions were counted and a mean value was obtained. Cardiomyocyte surface area was determined from sections of the left ventricular myocardium stained with haematoxylin and eosin or wheat germ agglutinin coupled to Alexa Flour 488 (1:100; Invitrogen, W11261). Images were analysed using the AxioVision (Zeiss) software packages. In vivo starvation experiments We performed in vivo starvation experiments as described earlier [45] with some modifications. For animals to be starved, we placed them in single cages with no access to food, but ad libitum access to water 3 h after the start of the light phase. Together with the animal ethics department, we established an ethically acceptable protocol for starvation using the published 'body condition scoring' criteria [46] , which showed a period of 31 h of starvation as maximally tolerable. Accordingly, we monitored all the starving mice during the experiment and evaluated their health status based on the change in following parameters: body weight, body condition, hydration condition, alertness and reaction to provocation, and body posture, locomotion and hair coat. After 31 h of starvation, mice were killed by cervical dislocation and heart tissues were isolated and processed as described for corresponding experiments. Quantitative RT–PCR analyses RNA was isolated using Trizol reagent (Invitrogen) from tissues or cultured cells. For quantitative detection of miRNA, TaqMan MiRNA assays (Applied Biosystems), iScript Select cDNA synthesis kit (Bio-Rad) and iQSupermix (Bio-Rad) kits were used according to the manufacturer's instructions. Rnu6b was used as control for normalization. For quantitative detection of mRNA levels, complementary DNAs were synthesized by using oligo-dT primers and iScript Select cDNA synthesis kit (Bio-Rad). Real-time PCR analyses were performed using specific set of primers and iQSYBR Green mix (Bio-Rad). Glyceraldehyde 3-phosphate dehydrogenase (GAPDH) levels were used for normalization of the gene-specific expression levels. MiRNA-1 expression levels were determined by a specific Taqman-RT-PCR kit for miR-1 (Applied Biosystems). Used oligonucleotide primer sequences are depicted in Supplementary Table S3 . Protein expression analyses Tissue or cells were lysed with 1× Cell lysis buffer (Cell Signaling) and protein isolation was done according to manufacturer's instructions. A measure 20–40 μg of protein was loaded on SDS–polyacrylamide gel electrophoresis gel for separation, which was followed by blotting of protein on polyvinylidene fluoride membrane in Mini Trans-Blot electrophoretic transfer cell (Bio-Rad). Afterwards, different antigens were detected using following primary antibodies: FoxO3 (1:1,000; Cell Signaling, #2,497), pAKT (1:500; Cell Signaling, #9,271), Akt (1:1,000; Cell Signaling, #9,272), LC3 (1:1,000; Abcam, ab48394), p62 (1:1,000; Abcam, ab56416), p-mTOR (1:500; Cell Signaling, #5,536), mTOR (1:1,000; Cell Signaling, #2,983), GFP (1:1,000; Abcam, ab1218) and GAPDH (1:10,000; Abcam, ab8245). HRP-conjugated secondary antibodies and luminol/paracumaric acid/H 2 O 2 is used for detection of the specific bands. Intensities of the obtained bands were quantified using ScionImage software. Calcineurin and NFAT assays Calcineurin assay was performed using Calcineurin Cellular Activity Assay Kit (Enzo Life Sciences) according to manufacturer's instructions. End-product quantification was done by measuring absorbance at 620 nm on a microplate reader (Synergy HT). For determination of NFAT activity, neonatal rat cardiomyocytes were seeded into 48-well plates and transfected after 24 h with a scrambled miR control, miR-132 and miR-212 (final concentration 50 nM; Ambion/Applied Biosystems, New Jersey, USA) using Lipofectamine 2000 (Invitrogen) according to the manufacturer's protocol. Cells were cultured for 24 h and NFAT luciferase reporter construct containing repetitive NFAT recognition sites (gift from J Molkentin, University of Cincinatti) was transfected as described above (final concentration: 0.75 ng μl −1 ). Forty-eight hours later the respective groups were stimulated with PE (50 μM) for 24 h. Luciferase activity was determined using Luciferase Assay System (Promega, Mannheim, Germany) and protein concentration was measured using the Pierce BCA Protein Assay Kit (Thermo Scientific, Bonn, Germany), both according to the manufacturer's protocol. Statistical analysis StatView and GraphPad prism software were used to perform unpaired Student's t -test in case of two treatment groups (data sets) or one-way ANOVA following Fisher's post-test analysis for more than two groups (data sets). For the Kaplan–Meier survival assay, the log-rank (Mantel-Cox) test was used. Further experimental methods used in this study are presented in the Supplementary Methods section in the Supplementary Information available online at www.nature.com/ncomms How to cite this article: Ucar, A. et al . The miRNA-212/132 family regulates both cardiac hypertrophy and cardiomyocyte autophagy. Nat. Commun. 3:1078 doi: 10.1038/ncomms2090 (2012).